Evidence for a material gradient in the adhesive tarsal setae of the ladybird beetleCoccinella septempunctata For an insect to be able to efficiently attach to surfaces, the adhesive pads on the distal parts of its legs must establish large contact areas. In case of hairy adhesive pads this requires flexibility of the contact-forming bristles, called adhesive tarsal setae. However, too flexible setae would have a low mechanical stability resulting in a decreased attachment ability of the pads. Here we show that the adhesive tarsal setae of the ladybird beetle Coccinella septempunctata feature pronounced gradients in the material composition and properties along their length. The Young’s modulus ranges from 1.2 MPa at the tips, where we found the incorporation of high proportions of the elastic protein resilin, to 6.8 GPa at the bases of the setae. These gradients likely represent an evolutionary optimization, which increases the performance of the adhesive system by enabling effective adaptation to rough surfaces while simultaneously preventing lateral collapse of the setae. Insect attachment organs, especially hairy adhesive pads, have long fascinated biologists [1] , [2] , [3] , and their morphology, ultrastructure and adhesion capabilities have been described in numerous studies [4] , [5] , [6] , [7] , [8] , [9] . The successful contact formation of such biological attachment systems depends on their ability to adapt to different surface topographies, which may be increased by various structural features. In hairy adhesive pads of insects, the hierarchical organization enables the formation of multiple contacts [10] and crack trapping mechanisms [11] providing advantages in the attachment to rough substrates. Adhesion is usually proportional to the area of real contact between two surfaces [12] . In this context, material flexibility is of great importance for the contact formation by adhesive systems because with a flexible material the potential real contact area between the adhesive system and a rough substrate can be increased. However, an increase in the attachment structures’ material flexibility may lead to a decrease of their mechanical stability. That is why in hairy adhesive pads contact-forming bristles, called adhesive tarsal setae, consisting of too soft material would buckle and cluster together very easily [13] , [14] resulting in a reduction of the contact stability and the functional advantages of the multiple contacts. Accordingly, the material properties of such setae represent an optimization problem. It is conceivable that during the evolution this problem has been solved by the presence of gradients in the material composition and the mechanical properties of the respective structures. Such gradients are well known for biological structures [15] and have previously been reported for smooth attachment devices of insects [16] . Pure bulk materials are almost absent in biological structures where proper combinations of different constituents often lead to mechanical gradients with important functional significances. This has, for example, been shown for insect cuticle [17] , snake skin [18] and human teeth [19] , [20] . The main goal of the present study was to analyse the material composition and the material properties of the adhesive tarsal setae of the ladybird beetle Coccinella septempunctata in detail to test the hypothesis of a material gradient being present within these setae. For the analyses, we applied atomic force microscopy (AFM) and confocal laser scanning microscopy (CLSM). Previous studies on other biological materials [21] , [22] , [23] have indicated that AFM nanoindentation is a well-suited method to analyse local mechanical properties of small volumes of the material of the adhesive tarsal setae. CLSM has been shown to have a great potential for visualizing the morphology and the material composition of arthropod exoskeleton structures with sub-micrometre resolution [24] making this technique ideal to evaluate a supposed material gradient within the adhesive tarsal setae. An influence of dehydration on the Young’s modulus of insect cuticle has repeatedly been reported [17] , [25] . Accordingly, dehydration might also change the material properties and thus the attachment ability of the adhesive tarsal setae. While the stiffness of a whole setal array within a beetle adhesive pad has already been analysed [26] , information on the correlation between the water content and the mechanical properties of the setal material is still missing. For this reason, our study also aimed at investigating this correlation by performing mechanical tests at the level of individual setae with both fresh and dried adhesive tarsal setae of C. septempunctata . In the framework of this study, we focused on analysing the adhesive tarsal setae of the second (the most distal) adhesive pad of female beetles’ forelegs. However, test analyses and measurements have shown that the material composition and the material properties of the adhesive tarsal setae described below are found in both adhesive pads of all three pairs of legs of C. septempunctata . Morphology and material composition of the adhesive tarsal setae Scanning electron microscopy (SEM) and CLSM revealed that the second adhesive pad of the forelegs of female C. septempunctata contains two types of adhesive tarsal setae, one being characterized by a widened spatula-like tip and the other by a pointed tip ( Fig. 1 ). Both setal types have tubular basal parts and are flattened towards their tips. Spatula-like setae are located only in the distal part of the adhesive pad, while the rest of the pad is covered by setae with pointed tips. In the proximal part of the pad, the setae have a length of about 50 μm. This length increases to about 80 μm towards the distal end of the pad. Non-adhesive setae located on the lateral and dorsal parts of the pad also feature lengths of about 50–80 μm, and they possess pronounced parallel longitudinal grooves. When being critical-point dried, the tips of the adhesive tarsal setae tend to bend ventrally. In the scanning electron microscope, the resulting preparations even tend to coil up in this direction when being exposed to the electron beam at an acceleration voltage of 10 kV ( Fig. 2 ). 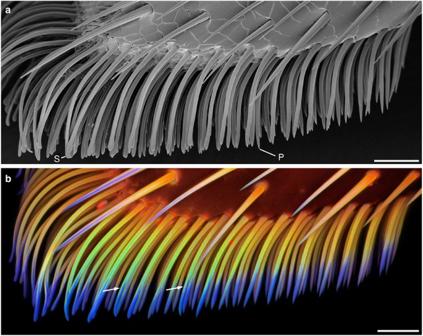Figure 1: Morphology and material composition of adhesive tarsal setae. Ventral part of the second adhesive pad of a foreleg of a femaleCoccinella septempunctata, lateral view. (a) Scanning electron micrograph (the specimen was dried using 1-propanol). (b) CLSM maximum intensity projection showing an overlay of the four different autofluorescences mentioned in the text. The arrows indicate the dorso-ventral material gradient in exemplary setae. S, exemplary spatula-like seta; P, exemplary seta with a pointed tip. Scale bars, 25 μm. Figure 1: Morphology and material composition of adhesive tarsal setae. Ventral part of the second adhesive pad of a foreleg of a female Coccinella septempunctata , lateral view. ( a ) Scanning electron micrograph (the specimen was dried using 1-propanol). ( b ) CLSM maximum intensity projection showing an overlay of the four different autofluorescences mentioned in the text. The arrows indicate the dorso-ventral material gradient in exemplary setae. S, exemplary spatula-like seta; P, exemplary seta with a pointed tip. Scale bars, 25 μm. 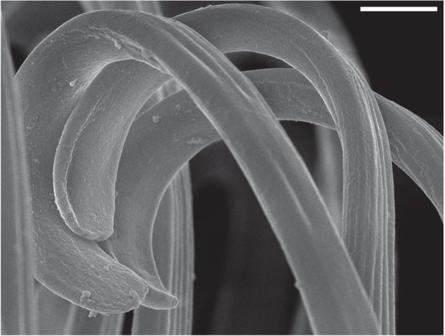Figure 2: Coiling up of adhesive tarsal setae. Scanning electron micrograph showing the tips of spatula-like adhesive tarsal setae of the second adhesive pad of a foreleg of a femaleCoccinella septempunctata. The coiling up of the setae occurred during the visualization of the preparation in the scanning electron microscope using an acceleration voltage of 10 kV. Scale bar, 2 μm. Full size image Figure 2: Coiling up of adhesive tarsal setae. Scanning electron micrograph showing the tips of spatula-like adhesive tarsal setae of the second adhesive pad of a foreleg of a female Coccinella septempunctata . The coiling up of the setae occurred during the visualization of the preparation in the scanning electron microscope using an acceleration voltage of 10 kV. Scale bar, 2 μm. Full size image Close to the tip, the diameter of the adhesive tarsal setae depends significantly on the hydration condition of the material. While dried setae feature diameters of 2.0±0.1 μm, fresh ones exhibit diameters of 2.2±0.3 μm ( P ≤0.005, one-way analysis of variance (ANOVA) (SigmaStat 3.5, Systat Software, Chicago, USA); the diameters were measured 5 μm proximally to the tip). In the basal part of the setae (35 μm from the tip), no diameter differences between fresh and dried samples were observed, which hints at a difference in the material composition between the tips and the bases of the setae. The CLSM analyses revealed the presence of considerable proportions of resilin in the adhesive tarsal setae, indicated by the blue autofluorescence of resilin [24] . At the tips of the setae, the material composition is strongly dominated by resilin, whereas the central and proximal parts of the setae mainly consist of other materials (other proteins and very likely mainly chitin), indicated by the dominance of green and red autofluorescences in these structures ( Fig. 1b ). The transition from the resilin-dominated distal parts to setal sections, which mainly consist of material other than resilin, is characterized by a rather pronounced longitudinal gradient found in a distance of about 15–20 μm from the setal tips. In the range of this gradient, a second gradient is present. The latter gradient is orientated in dorso-ventral direction and features higher resilin concentrations in the ventral part, facing the substrate during contact formation, and lower resilin concentrations in the dorsal part of each seta (see arrows in Fig. 1b ). Material properties of the adhesive tarsal setae Before the AFM nanoindentations, AFM images of the adhesive tarsal setae were made to verify the setal type (spatula-like or with pointed tips) to be indented ( Fig. 3 ). As the non-adhesive setae ( Fig. 3g–i ) most probably have no attachment function, only spatula-like setae ( Fig. 3a–c ) and setae with pointed tips ( Fig. 3d–f ) were used for the indentation measurements. 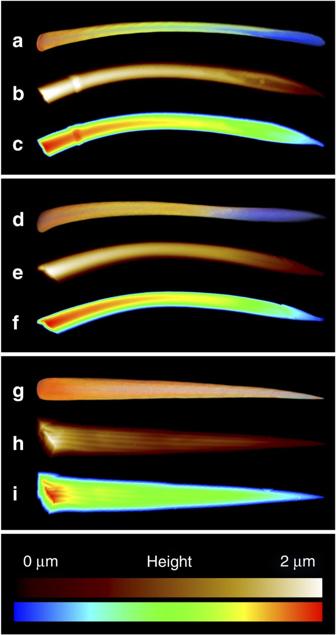Figure 3: Overview of tarsal setae. Comparison of results from CLSM (a,d,g) and AFM ((b,e,h) height mode; (c,f,i) hi-low structure mode) analyses of adhesive ((a–c) spatula-like; (d–f) with pointed tips) and non-adhesive (g–i) tarsal setae of the second adhesive pad of forelegs of femaleCoccinella septempunctata. The confocal laser scanning micrographs indicate the presence of a pronounced longitudinal material gradient in the adhesive tarsal setae with high concentrations of resilin (blue) in the setal tips. The AFM height images give a good impression of the overall geometry of the setae, while the AFM images obtained with the hi-low structure mode emphasize small structural differences (especially at the setal tips) not distinguishable in the height images. The confocal laser scanning micrographs show details fromFig. 1b. Figure 3: Overview of tarsal setae. Comparison of results from CLSM ( a , d , g ) and AFM (( b , e , h ) height mode; ( c , f , i ) hi-low structure mode) analyses of adhesive (( a – c ) spatula-like; ( d – f ) with pointed tips) and non-adhesive ( g – i ) tarsal setae of the second adhesive pad of forelegs of female Coccinella septempunctata . The confocal laser scanning micrographs indicate the presence of a pronounced longitudinal material gradient in the adhesive tarsal setae with high concentrations of resilin (blue) in the setal tips. The AFM height images give a good impression of the overall geometry of the setae, while the AFM images obtained with the hi-low structure mode emphasize small structural differences (especially at the setal tips) not distinguishable in the height images. The confocal laser scanning micrographs show details from Fig. 1b . Full size image The measurements performed on individual adhesive tarsal setae showed a gradient of the Young’s modulus over the entire setal length in fresh samples ( Fig. 4a ) as well as a statistically significant difference between the material properties of fresh and dried samples (described below). A statistically significant difference in the Young’s modulus between spatula-like setae and setae with pointed tips was not found ( P =0.976, H =21.954, 37 degrees of freedom (DOF), one-way ANOVA on ranks, Kruskal–Wallis post-hoc test), and thus the results obtained from both setal types were pooled together for subsequent analyses. 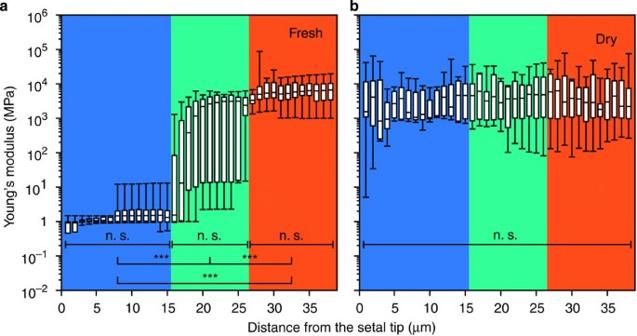Figure 4: Young’s modulus of fresh and dried adhesive tarsal setae. Box-and-Whisker plots showing the median (n=50) Young’s modulus of fresh (a) and dried (b) adhesive tarsal setae of the second adhesive pad of forelegs of femaleCoccinella septempunctataobtained by 38 AFM nanoindentations (1 μm spacing) along each seta. The borders of the boxes define the 25th and 75th percentiles, the median is indicated by a horizontal line, and the error bars define the 10th and 90th percentiles (n. s.=not significant, ***=highly significant). The background colours indicate the different seta sections. Figure 4: Young’s modulus of fresh and dried adhesive tarsal setae. Box-and-Whisker plots showing the median ( n =50) Young’s modulus of fresh ( a ) and dried ( b ) adhesive tarsal setae of the second adhesive pad of forelegs of female Coccinella septempunctata obtained by 38 AFM nanoindentations (1 μm spacing) along each seta. The borders of the boxes define the 25th and 75th percentiles, the median is indicated by a horizontal line, and the error bars define the 10th and 90th percentiles (n. s.=not significant, ***=highly significant). The background colours indicate the different seta sections. Full size image In fresh setae, the median value of the Young’s modulus of the material in the distal most section, between 0 and 15.5 μm from the tip, is low (1.2±0.3 MPa). Compared with this, the median value of the Young’s modulus of the material located between 15.5 and 26.5 μm from the tip (transition zone) is significantly higher (2.43±1.9 GPa). Between this transition zone and the setal base, the Young’s modulus reaches its maximum value of 6.8±1.2 GPa. The differences in the Young’s modulus between the three sections analysed are statistically highly significant ( P ≤0.001, one-way ANOVA on ranks, Kruskal–Wallis post-hoc test), whereas within each section no statistical difference was found ( P 1 =0.084, H 1 =19.193, 14 DOF; P 2 =0.884, H 2 =3.010, 10 DOF; P 3 =0.769, H 3 =7.364, 11 DOF; one-way ANOVA on ranks, Kruskal–Wallis post-hoc test) ( Fig. 4a ). In dried setae, the Young’s modulus exhibits no statistically significant differences along the entire setal length ( P =0.999, H =15.781, 37 DOF, one-way ANOVA on ranks, Kruskal–Wallis post-hoc test) ( Fig. 4b ). The median value of the Young’s modulus (7.2±1 GPa) of dried setae is slightly higher than that measured at the stiff basal part of fresh setae (6.8±1.2 GPa). Compared with the tips of the fresh setae, the Young’s modulus of the tips of the dried setae features a statistically highly significant difference ( P ≤0.001, one-way ANOVA on ranks, Kruskal–Wallis post-hoc test), while such a difference does not exist between the basal parts of the fresh and the dried setae ( P =0.244, H =1.356, 1 DOF, one-way ANOVA on ranks, Kruskal–Wallis post-hoc test). The pronounced differences in the material properties between the tips and the bases of fresh adhesive tarsal setae are, in addition to the Young’s modulus values, reflected by the behaviour of the respective materials during the AFM nanoindentations. In the typical force-distance curve (FDC) obtained from the material of the setal tips, the points of zero indentation of the approach (loading) and retraction (unloading) parts are at the same location ( Fig. 5a ). By contrast, the typical FDC obtained from the material of the setal bases features approach and retraction parts with zero points, which are shifted against each other along the x -axis ( Fig. 5b ). This indicates that the material in the tips exhibits only elastic deformation, while the material in the bases features both elastic and, to some extent, plastic deformation. 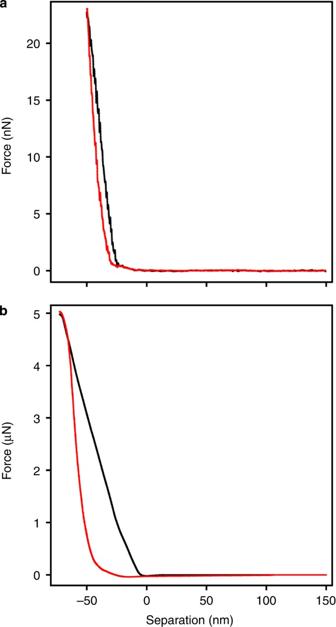Figure 5: FDCs obtained by AFM nanoindentation. Exemplary FDCs from nanoindentations of the setal material located 4 μm proximally to the tip (a) and in the base (36 μm from the tip) (b) of a fresh adhesive tarsal seta. The black lines represent the approach parts of the curves, and the red lines illustrate the retraction parts. Figure 5: FDCs obtained by AFM nanoindentation. Exemplary FDCs from nanoindentations of the setal material located 4 μm proximally to the tip ( a ) and in the base (36 μm from the tip) ( b ) of a fresh adhesive tarsal seta. The black lines represent the approach parts of the curves, and the red lines illustrate the retraction parts. Full size image The results of the present study clearly show that the adhesive tarsal setae of C. septempunctata are composite structures exhibiting two pronounced longitudinal gradients in the material composition and the material properties. Both gradients have a similar spatial distribution indicating that they are related to each other. Compared with sclerotized chitinous exoskeleton material, the protein resilin, which we found to be present in high proportions within the tips of the adhesive tarsal setae, is soft, flexible and elastic [27] , [28] , [29] , [30] . Accordingly, the low Young’s modulus values measured for the fresh setal tips are very likely caused by the high proportions of resilin within the tips. The presence of resilin has previously been reported for a large variety of arthropod exoskeleton structures, and numerous resilin functions such as generating flexibility, providing fatigue and wear resistance and storing energy for high-speed movements have been described [27] , [29] , [30] , [31] , [32] , [33] , [34] , [35] . We hypothesize that the high proportions of resilin in the setal tips have two main functions described in the following. Previous studies have shown a strong relationship between the contact area of adhesive structures and their adhesion capabilities [36] , [37] . In this context, the presence of high resilin proportions likely allows for ideal properties of the setal tips. It is conceivable that the resilin-dominated tips have a large potential for an effective adaptation to rough substrates due to their softness and flexibility and therefore may enable the formation of a larger contact area. By contrast, the relatively stiff material in the middle and basal sections of the setae may have the function to provide a uniform stress distribution during the detachment of the adhesive pad and to prevent buckling and condensation of the setae. The differences in the stiffness between different materials present in the setae are vividly reflected in the setal tips’ tendency to bend or even coil up when being dried and exposed to a relatively energy-rich electron beam. In this context, the fact that the setae bend or coil up in the ventral direction, which is responsible for the contact formation with the substrate, suggests that the ventral setal parts contain the highest resilin proportions. This is in accordance with the CLSM results indicating the presence of a second gradient of the material composition orientated in dorso-ventral direction. The bending and coiling up of the setae may be caused by the different hydration states of resilin (highly hydrated) and chitinous material (less hydrated). During drying, the material with higher resilin proportions very likely undergoes a more pronounced shrinkage resulting in the setae behaving like a bimetal stripe and being bent or coiled up ventrally. In addition, because of the resilin’s fatigue and wear resistance previously observed in several arthropod exoskeleton structures such as beetle wings [34] , the high resilin proportions in the tips of the adhesive tarsal setae may turn the hairy adhesive pads into durable attachment systems, which are unsusceptible to abrasion also when being used on rough substrates. This is of utmost importance for the beetles as they need to sustain their attachment performance for a high number of movement cycles during lifelong locomotion. The Young’s moduli measured in the present study correspond well to previously published values for insect cuticle [28] . Furthermore, our results, showing that the Young’s modulus of the setal tip material strongly increases from 1.2 MPa in the hydrated situation to 7.2 GPa in the dehydrated one, are in accordance with earlier observations indicating that the material properties of resilin strongly depend on its hydration status, which is due to the fact that proteins are plasticized by water [28] , [29] . Under natural conditions, resilin is very likely always hydrated [28] . Beetles are known to produce tarsal liquids, which have been assumed to contribute to the adhesion capabilities by means of capillary processes [38] , [39] and cleaning effects [40] , [41] . Based on our assumption that the presence of high resilin concentrations in the setal tips increases the attachment ability of the adhesive pads, it becomes obvious that the hydration of resilin may be essential for keeping the attachment performance of the beetles on a high level. In this context, it is imaginable that the beetles’ tarsal liquids, which evaporate relatively slowly [42] , have the function to cover the setae and thereby maintain the hydration of the resilin in the setal tips. In conclusion, this study has revealed for the first time the presence of high proportions of resilin in the tips of the adhesive tarsal setae of C. septempunctata and pronounced gradients in the material composition and the material properties within these setae. These setal features very likely have the function to enhance the adhesive pads’ ability for contact formation and prevention of setal condensation resulting in an increased attachment performance of C. septempunctata . The structural characteristics of this beetle species’ adhesive pads and their functional significance may represent an adaptation to living on rough substrates. Sample collection and preparation For all analyses and measurements, fresh forelegs of C. septempunctata females, collected in the botanical garden of the university in Kiel, Germany, were used. For the CLSM analyses, the beetles were frozen at −70 °C, and later the legs were removed as described earlier [24] . The beetles used for all other analyses and measurements were kept in plastic boxes on clean moist paper towels to prevent leg contamination and animal desiccation. For leg preparation, the beetles were anesthetized in a jet of CO 2 , and the forelegs were cut off using a razor blade. SEM imaging To properly verify the structures visible on the CLSM and AFM images, scanning electron micrographs showing the second adhesive pad of the beetle legs were made. For this purpose, fresh legs were dehydrated in a graded series of ethanols (Carl Roth GmbH Co. KG, Karlsruhe, Germany; 70, 80, 90, 96% and two times 100%, 15 min each) and dried for 12 h in an exsiccator using 1-propanol (Sigma-Aldrich Chemie GmbH, Steinheim, Germany) as previously described [43] . In addition, a few dehydrated legs were critical point dried using a Polaron E3000 critical point dryer (QuorumTechnologies Ltd, East Grinstead, UK). The dried specimens were mounted and sputter-coated as described in an earlier study [43] and visualized in a Hitachi S-4800 field emission scanning electron microscope (Hitachi High-Technologies Corporation, Tokyo, Japan) at an acceleration voltage of either 5 kV or 10 kV and an emission current of 10 μA applying a mixture of the upper (detection of high-angle secondary electrons) and the lower (detection of low-angle secondary electrons) detector. CLSM imaging Fresh beetle forelegs were transferred to glycerine (≥99.5%, free of water, two times distilled, Carl Roth GmbH & Co. KG) and mounted using high-precision cover slips (thickness=0.170 mm±0.005 mm, refractive index=1.52550±0.00015, Carl Zeiss Microscopy GmbH, Jena, Germany) as described earlier [24] . The presence and the distribution of four different autofluorescences within the second adhesive pad of the legs were analysed using the confocal laser scanning microscope Zeiss LSM 700 (Carl Zeiss Microscopy GmbH) equipped with an upright microscope (Zeiss Axio Imager.M1m) and four solid-state lasers (wavelengths: 405, 488, 555, 639 nm) and applying a previously described method [24] . In contrast to this method, instead of a longpass emission filter transmitting light with wavelengths ≥560 nm, a longpass emission filter transmitting light with wavelengths ≥640 nm was used to detect the autofluorescence excited by 639 nm. However, this did not have any influence on the results. For the visualization, a 20 x objective (Zeiss Plan-Apochromat, air immersion, numerical aperture=0.8, Carl Zeiss Microscopy GmbH) was used. AFM imaging and nanoindentation Immediately after separation, the legs of 10 beetles were dipped into liquid nitrogen, and the frozen tarsal setae were separated from the second adhesive pad by scraping using a deeply frozen razor blade. The truncated setae were fixed to an object slide by a thin layer of Leica CV Mount (Leica Instruments GmbH, Nussloch, Germany). The material properties of two types of adhesive tarsal setae (spatula-like or with pointed tips) were analysed by AFM nanoindentation. These setal types are the dominant ones present in both sexes of C. septempunctata . To verify the setal type to be measured, images of each seta were recorded before indentation. Non-adhesive setae located on the dorsal and lateral sides of the adhesive pad were also imaged for comparison but not indented. To evaluate the effect of dehydration on the Young’s modulus of the adhesive tarsal setae, the samples were divided into two groups (five beetles per group). The setae of the first group were imaged and indented immediately after the preparation, whereas the setae of the second group were dried in an exsiccator for 72 h before the analyses. A NanoWizard® scanning probe microscope (SPM) (JPK Instruments, Berlin, Germany), mounted on an inverted light microscope (Zeiss Axiovert 135, Carl Zeiss Microscopy GmbH) operated in the phase contrast mode, was used for imaging and nanoindentation. The high-frequency intermittent contact mode was applied to visualize the setae before indentation to be able to select specific sites. NanoWizard SPM® software 4.0.31 (JPK Instruments) was used to obtain AFM images and FDCs. All visualizations and nanoindentations of the first group of preparations (fresh setae) were performed in water (21 °C) to prevent desiccation during the analyses, while the preparations of the second group (dried setae) were imaged and indented in air under ambient laboratory conditions (relative humidity=30%, temperature=24 °C) ( Fig. 6 ). 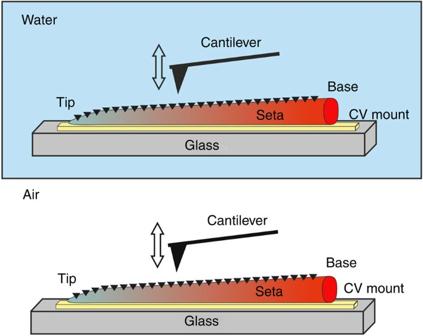Figure 6: AFM nanoindentation set-up. Schematic drawing of the set-up used for the AFM nanoindentations of the adhesive tarsal setae. The fresh setae were indented in a water basin. For the nanoindentation of the dried setae, the general set-up was identical but the setae were indented in air under ambient laboratory conditions. Figure 6: AFM nanoindentation set-up. Schematic drawing of the set-up used for the AFM nanoindentations of the adhesive tarsal setae. The fresh setae were indented in a water basin. For the nanoindentation of the dried setae, the general set-up was identical but the setae were indented in air under ambient laboratory conditions. Full size image Image acquisition in water and air was performed using high-frequency tapping mode cantilevers (NCH, NanoSensors, Neuchatel, Switzerland) at a scan rate of 0.5 Hz and an image size of 1024 × 1024 pixels. For the nanoindentation analyses, an indentation depth of 50 nm was used. This depth equates only about 2.5% of the thickness of the indented adhesive tarsal setae. Accordingly, any potential influence of the subjacent substrate on the determination of the Young’s modulus was definitely excluded. The spring constant (25 Nm −1 ) and the tip radius (10 nm) of the cantilever were ascertained before the analyses using the thermal noise method [44] and calibration grids, respectively. A comparison between the effective curvature radius of the cantilever tip and the setal tip (curvature radius=5.9 μm) and the effective curvature radius of the cantilever tip and the setal base (curvature radius=2.9 μm) yielded a difference of 1%. Accordingly, the influence of the setal morphology and the setal topography on the AFM nanoindentation results was negligible. Because the indented adhesive tarsal setae (both spatula-like and with pointed tips) featured a roughness mean square of 6.2 nm, the influence of the surface roughness was also negligible. A total of 38 sites located along the longitudinal axis of each seta were indented. In each case, the distance between two neighbouring sites was ~1 μm ( Fig. 6 ). Overall, images and nanoindentations of 100 adhesive tarsal setae (50 fresh and 50 dried, 10 setae per beetle, 5 beetles per group, 2 groups) were analysed. The Young’s modulus of the setae was calculated by fitting the initial portion of the retraction part of the FDCs [45] . Scanning probe image processing software version 5.1.2 (SPIP, Image Metrology A/S, Hørsholm, Denmark) was applied to fit the data, and SigmaStat 3.5 (Systat Software) was used to evaluate statistical differences between different samples. The Hertz contact model [46] is an approximation to the contact and very shallow indentation of two spheres, which are in contact. In the AFM literature, however, this term is often used to refer to a family of different models, which have been adapted for simple indentation geometries [47] , [48] , [49] , [50] . Test measurements performed at the beginning of our study clearly indicated that the material of the adhesive tarsal setae is not adhesive. Other than the official scientific term suggests the setae are not adhesive themselves. They enable adhesion due to contact splitting, adaptability and proper movement of the leg. For this reason, the application of the Hertz contact model is suited for the type of indentation measurements performed in our study [51] . Besides this, there are other reasons for our decision to apply the Hertz contact model. First, the initial portion of the retraction part of all FDCs obtained in our study was nearly linear. In such a case, the Hertz contact model is applicable [45] . In addition, this model is generally valid for indentation measurements conducted with both the circular paraboloid-shaped indenter tip and the small indentation depth used in our study [52] , [53] . Based on the application of the Hertz contact model, we determined the Young’s modulus, as previously described [54] , by with F being the force obtained from the FDCs, E the Young’s modulus, v the assumed Poisson ratio set to 0.5, R c the radius of the curvature of the cantilever tip (10 nm) and δ the indentation depth of 50 nm. How to cite this article: Peisker, H. et al. Evidence for a material gradient in the adhesive tarsal setae of the ladybird beetle Coccinella septempunctata . Nat. Commun. 4:1661 doi: 10.1038/ncomms2576 (2013).